Bmi1 limits dilated cardiomyopathy and heart failure by inhibiting cardiac senescence Dilated cardiomyopathy (DCM) is the most frequent cause of heart failure and the leading indication for heart transplantation. Here we show that epigenetic regulator and central transcriptional instructor in adult stem cells, Bmi1, protects against DCM by repressing cardiac senescence. Cardiac-specific Bmi1 deletion induces the development of DCM, which progresses to lung congestion and heart failure. In contrast, Bmi1 overexpression in the heart protects from hypertrophic stimuli. Transcriptome analysis of mouse and human DCM samples indicates that p16 INK4a derepression, accompanied by a senescence-associated secretory phenotype (SASP), is linked to severely impaired ventricular dimensions and contractility. Genetic reduction of p16 INK4a levels reverses the pathology of Bmi1-deficient hearts. In parabiosis assays, the paracrine senescence response underlying the DCM phenotype does not transmit to healthy mice. As senescence is implicated in tissue repair and the loss of regenerative potential in aging tissues, these findings suggest a source for cardiac rejuvenation. Dilated cardiomyopathy (DCM) is the commonest form of non-ischaemic cardiomyopathy and can lead to sudden cardiac death and heart failure [1] . The health burden associated with DCM is a major contribution to health-care costs; however, the mechanisms underlying the regulation of noninherited DCM remain unexplored [2] . DCM is defined by the presence of dilated and poorly functioning left ventricle in the absence of abnormal loading conditions, such as valve defect or hypertension or ischaemic heart failure sufficient to induce global systolic impairment. A large number of cardiac and systemic diseases can cause systolic impairment and left ventricular dilatation; however, in the majority of patients no identifiable cause is found (hence, idiopathic DCM). Therefore, understanding the aetiology of idiopathic DCM is of great clinical relevance in view of the devastating consequences of this disease in a large patient population. The epigenetic signature establishes a cell-type-specific chromatin pattern that is of paramount importance for cell commitment and regeneration during development and adulthood [3] , [4] , [5] . Epigenetic regulation offers a critical means for governing cardiac gene expression under different physiological and pathological states [6] . In fact, the nature of cardiomyopathy and heart failure intensely links with irregular cardiac gene expression. One of the causes of congenital heart disease is deficiency for specific epigenetic instructors during cardiogenesis [5] , such as the histone methyltransferases Ezh2 (ref. 7 ) and MLL2 (ref. 8 ), or transcription factors Tbx5 and Nkx2 -5 that require histone-modifying enzymes to regulate gene expression [5] . Essential epigenetic changes at developmental cardiac-specific genes are also required for reprogramming of cardiac fibroblasts (FBs) into cardiomyocytes (CMs) and for cardiac lineage commitment [9] , [10] . However, the role of critical epigenetic modifications in adult cardiac function has received comparatively little attention. A good example of that is the well-established role of epigenetic Bmi1 factor in the maintenance of adult stem cell populations [11] ; however, its direct or indirect implication in regulating the cardiac function is unknown. Senescence protects organisms against damaged cells by inducing a stable growth arrest not only in tumour suppression [12] but also in noncancer pathologies [13] . Growth arrest is achieved, at least in part, through activation of the p16 INK4a /Retinoblastoma tumour-suppressor pathways [14] , [15] . Concomitant with this arrest, senescent cells communicate with their environment, secreting a complex mixture of factors called the senescence-associated secretory phenotype (SASP) or senescence-messaging secretome [16] , [17] . Here we reasoned that the epigenetic factor Bmi1 might be involved in the maintenance of adult cardiac function. Using a combination of conditional knockout models, biochemical analysis, parabiotic assays and characterization of the DCM transcriptional signature in humans and mice, this study reveals the importance of a genuinely protective role of the epigenetic Bmi1 in cardiac adult pathophysiology, namely protection of adult heart from cellular senescence. Therefore, controlling cardiac gene expression by epigenetic-regulating factors gives a promising approach to the treatment of human cardiomyopathy. Bmi1 expression is not required for cardiogenesis Several epigenetic Polycomb regulators are differently regulated during embryonic development and adult aging [18] , prompting us to analyse endogenous cardiac Bmi1 expression in the mouse. The amount of Bmi1 increased progressively throughout cardiogenesis, stabilizing in adulthood, and then declining in the hearts of aged mice ( Supplementary Fig. 1a ). This profile correlated inversely with the levels of p16 INK4a ( Supplementary Fig. 1b ), as noted in other studies with adult stem cells [19] , [20] , [21] , [22] , [23] , [24] . To analyse the implication of Bmi1 in heart failure, we induced hypertrophy in wild-type mouse hearts, either surgically with a transverse aortic constriction (TAC) or by infusion with isoproterenol ( Supplementary Fig. 1c ). We additionally analysed the left ventricular myocardium from eight non-failing and eight failing human hearts. In humans and mice, analysis of cardiac Bmi1 expression showed a marked reduction in failing hearts, levels inversely correlated with p16 INK4a expression ( Supplementary Fig. 1c,d ). These results indicate a possible association of Bmi1 downregulation with the development of cardiac hypertrophy. To explore the implication of Bmi1 in cardiogenesis, we crossed Bmi1 fl/fl mice with Nkx2.5-Cre tg/+ mice [25] to induce cardiac-specific Bmi1 deletion from embryonic day (E) 7.5 onwards. Bmi1 f/f ;Nkx-Cre tg/+ mice were born at normal Mendelian frequency and were able to support pregnancy. Histologic examination of Bmi1 f/f ;Nkx-Cre tg/+ embryos at E14.5−E18.5 did not reveal any cardiac abnormality ( Fig. 1a ). Expression of Bmi1 mRNA on post-natal day 2 (P2) was significantly lower in Bmi1 f/f ;Nkx-Cre tg/+ hearts than in controls and correlated with below-normal levels of the epigenetic mark H3K9me3 ( Fig. 1b ; Supplementary Fig. 1e ). Interestingly, Bmi1 f/f ; Nkx-Cre tg/+ hearts also had a significantly higher heart-to-body-weight (HW/BW) ratio, and expressed higher levels of fetal cardiac genes than littermate controls ( Fig. 1c ; Supplementary Fig. 1f ). Histological comparison with Bmi1 f/f ;Nkx-Cre +/+ controls at 22 weeks after birth showed that Bmi1 -null hearts were enlarged and presented fibrosis and CMs with the above-normal cross-sectional area ( Fig. 1d ; Supplementary Fig. 1g ). Two-dimensional echocardiography revealed the hearts of Bmi1 f/f ; Nkx-Cre tg/+ mice to be dilated and poorly contractile ( Fig. 1e ). These hearts, moreover, had a markedly enlarged left ventricular internal diameter at diastole and severely depressed left ventricular mass and fractional shortening, a direct measure of cardiac contractile function, consistent with progressive DCM ( Fig. 1e,f ). Lung weight in 22-week-old Bmi1 f/f ;Nkx-Cre tg/+ mice was significantly increased ( Fig. 1g ; Supplementary Fig. 1h ), suggesting the development of lung oedema secondary to the LV dysfunction. This was confirmed by serial pulmonary magnetic resonance imaging (MRI), which revealed significant pulmonary congestion and oedema ( Fig. 1h ) coinciding with the impaired cardiac contractile function and maximal left ventricular dilatation for Bmi1-null hearts ( Fig. 1f ). Perl’s Prussian blue staining on lung sections revealed impaired permeability of the alveolar septal barrier in Bmi1 f/f ;Nkx-Cre tg/+ mice, indicated by the accumulation of siderophages (hemosiderin-laden macrophages) in the perivascular regions of Bmi1 f/f ;Nkx-Cre tg/+ lungs ( Fig. 1i ). All Bmi1 f/f ;Nkx-Cre tg/+ mice died between 20 and 30 weeks, whereas Bmi1 f/f ; Nkx-Cre +/+ had a normal lifespan ( Fig. 1j ). These data thus suggest that cardiac Bmi1 deletion during embryogenesis does not affect cardiogenesis but causes DCM in adulthood. 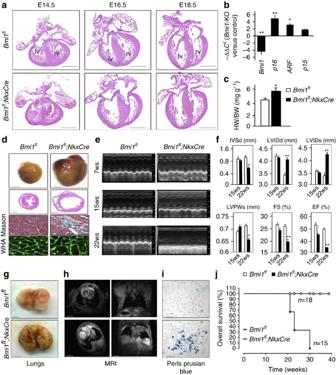Figure 1: Bmi1 is not required for normal cardiac development. (a) Representative heart sections fromBmi1f/f;Nkx-Cretg/+(Bmi1fl;NkxCre) andBmi1f/f;Nkx-Cre+/+(Bmi1f/) E14.5, E16.5 and E18.5 embryos (scale bar, 200 μm). Rv, right ventricle; lv, left ventricle. (b) Quantitative RT–PCR (qRT–PCR) analysis ofBmi1,p16INK4a,ARFandp15INK4bmRNA expression in total heart cells fromBmi1fl;NkxCre(Bmi1-knock out) mice. Data are standardized to β-actin levels and are expressed relative toBmi1f/(Control) mice (means±s.d.;n=12, *P<0.05; Student’st-test). (c) HW/BW ratio in 22-week-oldBmi1fl;NkxCremice andBmi1f/controls (means±s.d.;n=12, *P<0.05; Student’st-test). (d) Gross cardiac phenotype of 22-week-oldBmi1fl;NkxCremice andBmi1f/controls. Representative views are shown of external anatomy (top row; bars, 0.5 cm) and haematoxylin and eosin (H&E) staining on sections in adult hearts (second row; bars, 1 mm), Masson’s trichrome staining to detect fibrosis (third row; bars, 40 μm) and left ventricular muscle sections stained with wheatgerm agglutinin (WGA; bottom row; bars, 10 μm). (e,f)Trans-thoracic M-mode echocardiographic and physiological analyses ofBmi1fl;NkxCreandBmi1f/mice. Panelishows representative traces fromBmi1fl;NkxCreandBmi1f/mice at 7, 15 and 22 weeks of age. IVSd, diastolic interventricular septal wall thickness; LVDd, diastolic left ventricular internal dimension; LVDs, systolic left ventricular internal dimension; LVPWd, diastolic left ventricular posterior wall thickness; FS, fractional shortening of left ventricle dimension; EF, ejection fraction; LVmass, left ventricular mass. Data are means±s.d. (n=12, **P<0.001, *P<0.05; Student’st-test). (g) Representative images of whole lungs from 12-week-oldBmi1fl;NkxCremice andBmi1f/littermates. Scale bars, 5 mm. (h) Thoracic magnetic resonance MRI of similar mice in transverse view, showing both heart and lungs (left), and in the coronal view (right). Scale bars, 2.5 mm. (i) Representative Perls iron staining of lung sections from mice as ing,h(bars, 30 μm). (j) Kaplan–Meier survival curve forBmi1fl;NkxCremice andBmi1f/littermates (means±s.d.,P<0.001; Student’st-test). Figure 1: Bmi1 is not required for normal cardiac development. ( a ) Representative heart sections from Bmi1 f/f ;Nkx-Cre tg/+ ( Bmi1 fl ;NkxCre ) and Bmi1 f/f ; Nkx-Cre +/+ ( Bmi1 f/ ) E14.5, E16.5 and E18.5 embryos (scale bar, 200 μm). Rv, right ventricle; lv, left ventricle. ( b ) Quantitative RT–PCR (qRT–PCR) analysis of Bmi1 , p16 INK4a , ARF and p15 INK4b mRNA expression in total heart cells from Bmi1 fl ;NkxCre (Bmi1-knock out) mice. Data are standardized to β-actin levels and are expressed relative to Bmi1 f/ (Control) mice (means±s.d. ; n =12, * P <0.05; Student’s t -test). ( c ) HW/BW ratio in 22-week-old Bmi1 fl ;NkxCre mice and Bmi1 f/ controls (means±s.d. ; n =12, * P <0.05; Student’s t -test). ( d ) Gross cardiac phenotype of 22-week-old Bmi1 fl ;NkxCre mice and Bmi1 f/ controls. Representative views are shown of external anatomy (top row; bars, 0.5 cm) and haematoxylin and eosin (H&E) staining on sections in adult hearts (second row; bars, 1 mm), Masson’s trichrome staining to detect fibrosis (third row; bars, 40 μm) and left ventricular muscle sections stained with wheatgerm agglutinin (WGA; bottom row; bars, 10 μm). ( e , f ) Trans -thoracic M-mode echocardiographic and physiological analyses of Bmi1 fl ;NkxCre and Bmi1 f/ mice. Panel i shows representative traces from Bmi1 fl ;NkxCre and Bmi1 f/ mice at 7, 15 and 22 weeks of age. IVSd, diastolic interventricular septal wall thickness; LVDd, diastolic left ventricular internal dimension; LVDs, systolic left ventricular internal dimension; LVPWd, diastolic left ventricular posterior wall thickness; FS, fractional shortening of left ventricle dimension; EF, ejection fraction; LVmass, left ventricular mass. Data are means±s.d. ( n =12, ** P <0.001, * P <0.05; Student’s t -test). ( g ) Representative images of whole lungs from 12-week-old Bmi1 fl ;NkxCre mice and Bmi1 f/ littermates. Scale bars, 5 mm. ( h ) Thoracic magnetic resonance MRI of similar mice in transverse view, showing both heart and lungs (left), and in the coronal view (right). Scale bars, 2.5 mm. ( i ) Representative Perls iron staining of lung sections from mice as in g , h (bars, 30 μm). ( j ) Kaplan–Meier survival curve for Bmi1 fl ;NkxCre mice and Bmi1 f/ littermates (means±s.d., P <0.001; Student’s t -test). Full size image Adult Bmi1 deficiency causes DCM To further test the contribution of Bmi1 deficiency to heart disease, we engineered CM-specific Bmi1 deletion in adulthood by crossing Bmi1 fl/fl mice [24] with the α -myosin heavy chain ( αMHC)-Cre tg/+ strain [26] . Conditional mutants occurred at a normal Mendelian ratio, indicating an absence of embryonic lethality. Examination of 5-week-old Bmi1 f/f ;αMHC-Cre tg/+ mice confirmed cardiac Bmi1 deletion ( Supplementary Fig. 2a ). At 12 weeks of age, Bmi1 f/f ;αMHC-Cre tg/+ mice showed typical features of DCM: impaired cardiac ejection fraction, a high HW/BW ratio, enlarged CMs, fibrosis and larger-than-normal ventricular chambers ( Fig. 2a,b ; Supplementary Fig. 2b ). These cardiac defects were accompanied by pulmonary oedema and the presence of siderophages ( Fig. 2c–e ). Consistent with this phenotype, adult Bmi1 f/f ;αMHC-Cre tg/+ mice developed full-blown DCM and suffered heart failure at 15–20 weeks of age ( Fig. 3f ). 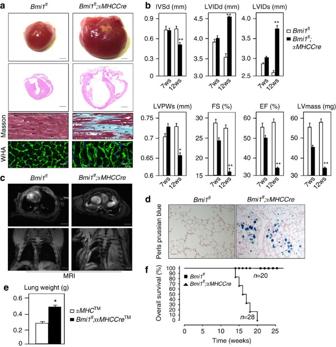Figure 2: Bmi1 activation blocks development of cardiac hypertrophy. (a) Gross cardiac phenotype ofBmi1fl;αMHCCremice andBmi1flcontrols. Representative views are shown of external anatomy and H&E staining on sections in adult hearts (12-week-old; top two rows; bars, 50 mm), Masson’s trichrome staining to detect fibrosis (third row; bars, 40 μm) and left ventricular muscle sections stained with WGA to detect cardiomyocyte borders (bottom row; bars, 10 μm). (b) M-mode echocardiographic analysis ofBmi1fl;αMHCCreandBmi1flmice. IVSd, diastolic interventricular septal wall thickness; LVDd, diastolic left ventricular internal dimension; LVDs, systolic left ventricular internal dimension; LVPWd, diastolic left ventricular posterior wall thickness; FS, fractional shortening of left ventricle dimension; EF, ejection fraction; LVmass, left ventricular mass. Data are means±s.d. (n=13, **P<0.001, *P<0.05; Student’st-test). (c) Thoracic MRI ofBmi1fl;αMHCCreandBmi1flmice in transverse view, showing both heart and lungs (top), and in coronal view (bottom). Scale bars, 2.5 mm. (d) Representative Perls iron staining of lung sections from representative 12-week-oldBmi1fl;αMHCCreandBmi1fllittermates (bars, 30 μm). (e) Lung weight in 12-week-oldBmi1f/f;αMHCTM-Cretg/+andBmi1+/+;αMHCTM-Cretg/+mice (means±s.d.;n=10, *P<0.05; Student’st-test). (f) Kaplan–Meier survival curve forBmi1fl;αMHCCremice andBmi1fllittermates (means±s.d.**P<0.001; Student’st-test). Figure 2: Bmi1 activation blocks development of cardiac hypertrophy. ( a ) Gross cardiac phenotype of Bmi1 fl ;α MHCCre mice and Bmi1 fl controls. Representative views are shown of external anatomy and H&E staining on sections in adult hearts (12-week-old; top two rows; bars, 50 mm), Masson’s trichrome staining to detect fibrosis (third row; bars, 40 μm) and left ventricular muscle sections stained with WGA to detect cardiomyocyte borders (bottom row; bars, 10 μm). ( b ) M-mode echocardiographic analysis of Bmi1 fl ;α MHCCre and Bmi1 fl mice. IVSd, diastolic interventricular septal wall thickness; LVDd, diastolic left ventricular internal dimension; LVDs, systolic left ventricular internal dimension; LVPWd, diastolic left ventricular posterior wall thickness; FS, fractional shortening of left ventricle dimension; EF, ejection fraction; LVmass, left ventricular mass. Data are means±s.d. ( n =13, ** P <0.001, * P <0.05; Student’s t -test). ( c ) Thoracic MRI of Bmi1 fl ;α MHCCre and Bmi1 fl mice in transverse view, showing both heart and lungs (top), and in coronal view (bottom). Scale bars, 2.5 mm. ( d ) Representative Perls iron staining of lung sections from representative 12-week-old Bmi1 fl ;α MHCCre and Bmi1 fl littermates (bars, 30 μm). ( e ) Lung weight in 12-week-old Bmi1 f/f ;α MHC TM -Cre tg/+ and Bmi1 +/+ ;α MHC TM -Cre tg/+ mice (means±s.d. ; n =10, * P <0.05; Student’s t -test). ( f ) Kaplan–Meier survival curve for Bmi1 fl ;α MHCCre mice and Bmi1 fl littermates (means±s.d. ** P <0.001; Student’s t -test). 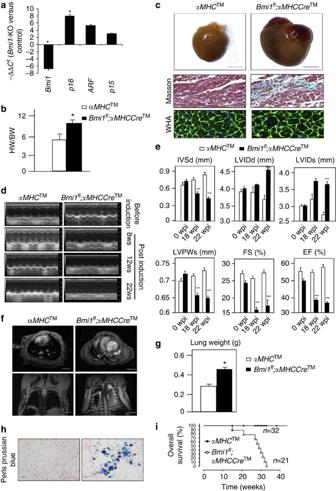Figure 3: Cardiac dysfunction in tamoxifen-treatedBmi1f/f;αMHCTM-Cretg/+mice. (a) qRT–PCR analysis of the mRNA expression ofBmi1,p16INK4a,ARFandp15INKbin total heart cells fromBmi1fl;αMHCCreTM(Bmi1-KO) andαMHCCreTM(Control) mice. Data are standardized to β-actin levels and are expressed relative to Control mice (means±s.d.;n=9, *P<0.05; Student’st-test). (b) HW/BW ratio inBmi1fl;αMHCCreTMmice andαMHCCreTMcontrols mice at 22 weeks post induction (27 weeks old; means±s.d.;n=10, *P<0.05; Student’st-test). (c) Gross cardiac phenotype ofBmi1fl;αMHCCreTMmice andαMHCCreTMcontrols at 22 weeks post induction (27 weeks old). Representative views are shown of external anatomy (bar, 50 mm), Masson’s trichrome staining to detect fibrosis (bars, 40 μm), left ventricular muscle sections stained with WGA to detect cardiomyocyte borders (bars, 10 μm). (d,e)Trans-thoracic M-mode echocardiographic and physiological analyses ofBmi1fl;αMHCCreTMandαMHCCreTMmice at 8, 12 and 22 weeks post induction. Paneleshows representative traces. Panelgshows echocardiographic measurements and physiological parameters. IVSd, diastolic interventricle septal wall thickness; LVDd, diastolic left ventricle internal dimension; LVDs, systolic left ventricle internal dimension; LVPWd, diastolic left ventricle posterior wall thickness; FS, fractional shortening of left ventricle dimension; EF, ejection fraction; LVmass, left ventricle mass. Data are means±s.d.;n=12, **P<0.001, *P<0.05; Student’st-test. (f) Thoracic MRI of representative 12-week-oldBmi1fl;αMHCCremice andBmi1f/flittermates in transverse view, showing both heart and lungs (top), and in coronal view (bottom). Scale bars, 2.5 mm. (g) Lung weight inBmi1fl;αMHCCreTMmice andαMHCCreTMcontrols at 22 weeks post induction (27 weeks old; means±s.d.;n=10, *P<0.05; Student’st-test). (h) Representative Perls iron staining of lung sections from representative 12-week-oldBmi1fl;αMHCCremice andBmi1f/flittermates (bars, 30 μm). (i) Kaplan–Meier survival curve forBmi1fl;αMHCCremice andBmi1f/flittermates (means±s.d. **P<0.001; Student’st-test). Full size image Figure 3: Cardiac dysfunction in tamoxifen-treated Bmi1 f/f ;αMHC TM -Cre tg/+ mice. ( a ) qRT–PCR analysis of the mRNA expression of Bmi1 , p16 INK4a , ARF and p15 INKb in total heart cells from Bmi1 fl ;αMHCCre TM (Bmi1-KO) and αMHCCre TM (Control) mice. Data are standardized to β-actin levels and are expressed relative to Control mice (means±s.d. ; n =9, * P <0.05; Student’s t -test). ( b ) HW/BW ratio in Bmi1 fl ;αMHCCre TM mice and αMHCCre TM controls mice at 22 weeks post induction (27 weeks old; means±s.d. ; n =10, * P <0.05; Student’s t -test). ( c ) Gross cardiac phenotype of Bmi1 fl ;αMHCCre TM mice and αMHCCre TM controls at 22 weeks post induction (27 weeks old). Representative views are shown of external anatomy (bar, 50 mm), Masson’s trichrome staining to detect fibrosis (bars, 40 μm), left ventricular muscle sections stained with WGA to detect cardiomyocyte borders (bars, 10 μm). ( d , e ) Trans -thoracic M-mode echocardiographic and physiological analyses of Bmi1 fl ;αMHCCre TM and αMHCCre TM mice at 8, 12 and 22 weeks post induction. Panel e shows representative traces. Panel g shows echocardiographic measurements and physiological parameters. IVSd, diastolic interventricle septal wall thickness; LVDd, diastolic left ventricle internal dimension; LVDs, systolic left ventricle internal dimension; LVPWd, diastolic left ventricle posterior wall thickness; FS, fractional shortening of left ventricle dimension; EF, ejection fraction; LVmass, left ventricle mass. Data are means±s.d. ; n =12, ** P <0.001, * P <0.05; Student’s t -test. ( f ) Thoracic MRI of representative 12-week-old Bmi1 fl ;αMHCCre mice and Bmi1 f/f littermates in transverse view, showing both heart and lungs (top), and in coronal view (bottom). Scale bars, 2.5 mm. ( g ) Lung weight in Bmi1 fl ;αMHCCre TM mice and αMHCCre TM controls at 22 weeks post induction (27 weeks old; means±s.d. ; n =10, * P <0.05; Student’s t -test). ( h ) Representative Perls iron staining of lung sections from representative 12-week-old Bmi1 fl ;αMHCCre mice and Bmi1 f/f littermates (bars, 30 μm). ( i ) Kaplan–Meier survival curve for Bmi1 fl ;αMHCCre mice and Bmi1 f/f littermates (means±s.d. ** P <0.001; Student’s t -test). Full size image To test whether heart failure was sensitive to the Bmi1 dosage, we analysed the hearts of Bmi fl/+ ;αMHC-Cre tg/+ and Bmi fl/+ ;αMHC-Cre +/+ mice. Young Bmi1 heterozygotes showed no noticeable cardiac defects ( Supplementary Fig. 2c ); however, at ~6 months, they developed characteristics of DCM, including a severely depressed ejection fraction ( Supplementary Fig. 2c ), a trend towards a high HW/BW ratio ( Supplementary Fig. 2d ) and interstitial fibrosis ( Supplementary Fig. 2e ). These mice invariably died by 7 months after birth ( Supplementary Fig. 2f ), indicating that Bmi1 is critical to maintain adult heart function. To confirm the requirement of Bmi1 in the adult heart, we used a tamoxifen (TM)-inducible α -myosin heavy chain ( αMHC) TM -Cre line [27] to delete Bmi1 in the hearts of 5-week-old adult mice ( Fig. 3a,b ). Heart weight and function in Bmi1 f/f ;αMHC TM -Cre tg/+ conditional knockouts and Bmi1 f/f ;αMHC TM -Cre +/+ and Bmi1 +/+ ;αMHC TM -Cre tg/+ control mice were monitored using histology and echocardiography ( Fig. 3c–e ). At 12 weeks post-TM treatment, average left ventricular internal diameter at diastole was similar in control and conditional knockout mice; however, dilatation and loss of contractility subsequently became evident in the mutants ( Fig. 3d,e ). At 22 weeks post induction, ventricular diameter in Bmi1 f/f ;αMHC TM -Cre tg/+ mice had increased from 3.8 mm at baseline to 4.59 mm, correlating with a fractional shortening of 17% ( Fig. 3d,e ). MRI revealed significant pulmonary congestion and oedema, which correlated with a 54% increase in lung weight, compared with TM-treated control littermates ( Fig. 3f,g ). Iron overload in the lung, detected by Perl’s staining, was also evident ( Fig. 3h ). TM-treated Bmi1 f/f ;αMHC TM -Cre tg/+ mice died between 28 and 32 weeks (23 and 27 weeks post induction), compared with only 1% of TM-treated control littermates ( Fig. 3i ). Thus, Bmi1 regulates CM function and maintenance throughout adult life. Bmi1 overexpression in the heart safeguarded the hypertrophic stage To assess the antihypertrophic effect of Bmi1, we crossed the doxycycline-inducible MLC2-rRTA tg/+ mouse line [28] with tetO-Bmi1 tg/tg mice, generating iBmi1 tg/tg ;MLC2 tg/+ mice and iBmi1 tg/tg ;MLC2 +/+ control littermates (hereafter iBmi1 tg ;MLC2 and iBmi tg control mice). Inclusion of doxycycline in the drinking water of 8-week-old iBmi1 tg/tg ;MLC2 tg/+ mice induced cardiac-specific overexpression of Bmi1 ( Fig. 4a ; Supplementary Fig. 3a ). Doxycycline treatment did not induce overt cardiac abnormalities in Bmi1 transgenic mice or control counterparts ( Fig. 4b–d ). As in wild-type mice, TAC surgery in doxycycline-treated iBmi1 tg/tg ;MLC2 +/+ controls triggered massive cardiac hypertrophy, an increase in CM cross-sectional area and fibrosis ( Fig. 4b–e ; Supplementary Fig. 3b ). In contrast, TAC surgery induced none of these symptoms in the hearts of doxycycline-treated iBmi1 tg/tg ;MLC2 tg/+ mice ( Fig. 4e ), indicating that Bmi1 overexpression blocks pathological ventricular remodelling. 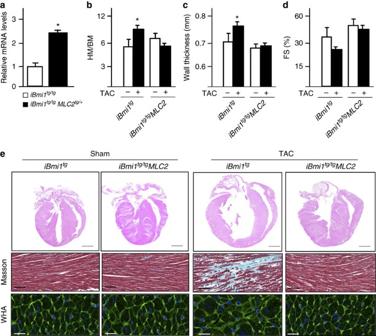Figure 4: Bmi1 activation blocks development of cardiac hypertrophy. (a) mRNA levels of Bmi1 in heart samples from nontransgenic control mice (iBmi1tg/tg) and Bmi1 transgenic mice (iBmi1tg/tg;MLC2tg/+; means±s.d.;n=8, *P<0.05; Student’st-test). (b) HW/BW ratios iniBmi1tg;MLC2mice andiBmitglittermates 4 weeks after the TAC surgery or sham operation. Data are means±s.d.;n=8 mice per group (means±s.d.;n=6, *P<0.05; Student’st-test). (c,d) Left ventricular wall thickness and fractional shortening measured using echocardiography in the same hearts as inb. (e) Representative low-magnification views of H&E-stained cross-sections at the midventricle from nontransgenic and Bmi1 transgenic mice subjected to sham or TAC treatment and stained with WGA (top; scale bars, 10 μm) or Masson’s trichrome to detect fibrosis (bottom; scale bars, 40 μm). Figure 4: Bmi1 activation blocks development of cardiac hypertrophy. ( a ) mRNA levels of Bmi1 in heart samples from nontransgenic control mice ( iBmi1 tg/tg ) and Bmi1 transgenic mice ( iBmi1 tg/tg ;MLC2 tg/+ ; means±s.d. ; n =8, * P <0.05; Student’s t -test). ( b ) HW/BW ratios in iBmi1 tg ;MLC2 mice and iBmi tg littermates 4 weeks after the TAC surgery or sham operation. Data are means±s.d. ; n =8 mice per group (means±s.d. ; n =6, * P <0.05; Student’s t -test). ( c , d ) Left ventricular wall thickness and fractional shortening measured using echocardiography in the same hearts as in b . ( e ) Representative low-magnification views of H&E-stained cross-sections at the midventricle from nontransgenic and Bmi1 transgenic mice subjected to sham or TAC treatment and stained with WGA (top; scale bars, 10 μm) or Masson’s trichrome to detect fibrosis (bottom; scale bars, 40 μm). Full size image Regulation of a cardiac-specific transcriptional programme by Bmi1 To explore the primary cause of DCM in Bmi1-null mice, we set out to identify differentially expressed genes by massively parallel sequencing of heart samples from DCM-diagnosed patients who had undergone heart transplant (hDCM) and from Bmi1 f/f ;αMHC TM -Cre tg/+ mice (17-week post induction; mDCM). Pairwise comparisons (with corresponding controls) identified 649 and 2,435 genes differentially expressed in mDCM and hDCM samples, respectively ( Fig. 5a ; Supplementary Data set ). Differentially upregulated genes common to mDCM and hDCM samples included those associated with the fetal cardiac gene programme [29] , such as Acta2 , Myh7 and Myl1 and genes encoding extracellular matrix components and regulators, such as Tgfβ , collagens, chemokines and metalloproteinases ( Fig. 5a ). Significantly upregulated senescence genes were the critical senescence regulator p16 INK4a ( Cdkn2a) [19] , [30] , [31] and essential components of the SASP (chemokines and Tgfβ family ligands; Fig. 5a ). Consistent with the proliferative arrest that accompanies senescence, we found downregulated genes related to cell-cycle progression such as CDKN3, CyclinD2 and CyclinA2 (CCNA2). There was, moreover, robust upregulation of genes encoding pro-inflammatory factors associated with the SASP, including interleukin (IL)-6, IL-7, granulocyte macrophage colony-stimulating factor and certain insulin-like growth factor-binding proteins [32] . These findings are suggestive of an important role of the senescence response mediated by the Bmi1/p16 INK4a axis in cardiac pathophysiology, consistent with the role of Bmi1 in preventing senescence in other contexts [19] . 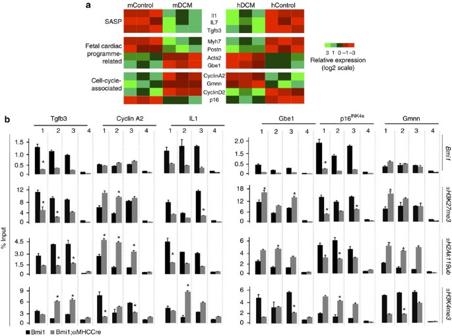Figure 5: Control of cardiac-specific profile by Bmi1. (a) Representative heat maps show the expression of genes with fetal cardiac programme-related genes, senescence-associated and cell-cycle functional annotations that are significantly down- and upregulated inBmi1f/f;αMHCTM-Cretg/+(mDCM) and control heart cells (mControl), and hDCM and hControl. The rows correspond to genes and the columns to samples. Gene expression values (relative to the mean expression in control cells) are indicated on a log2scale according to a colour scheme shown. (b) ChIP analyses of the promoter regions in the indicated genes from total heart cells fromBmi1f/f;αMHCTM-Cretg/+mice and littermate controls. Chromatin-bound DNA was probed with antibodies to Bmi1, H3K27me3, H2AK119 and H3K4me3. Percentages of input DNA are shown as the means±s.d. of triplicate independent experiments (*P<0.05; Student’st-test; Student’st-test). Figure 5: Control of cardiac-specific profile by Bmi1. ( a ) Representative heat maps show the expression of genes with fetal cardiac programme-related genes, senescence-associated and cell-cycle functional annotations that are significantly down- and upregulated in Bmi1 f/f ;αMHC TM -Cre tg/+ (mDCM) and control heart cells (mControl), and hDCM and hControl. The rows correspond to genes and the columns to samples. Gene expression values (relative to the mean expression in control cells) are indicated on a log 2 scale according to a colour scheme shown. ( b ) ChIP analyses of the promoter regions in the indicated genes from total heart cells from Bmi1 f/f ;αMHC TM -Cre tg/+ mice and littermate controls. Chromatin-bound DNA was probed with antibodies to Bmi1, H3K27me3, H2AK119 and H3K4me3. Percentages of input DNA are shown as the means±s.d. of triplicate independent experiments (* P <0.05; Student’s t -test; Student’s t -test). Full size image To assess the epigenetic signature on the promoter regions of Bmi1 target genes, chromatin silencing was examined by measuring ubiquitination of histone H2A at the Lys119 residue (H2AK119ub), a histone modification mediated by PRC1 (ref. 3 ), and by Bmi1-specific binding using mDCM and control hearts ( Fig. 5b ). Additional Ezh1/Ezh2-dependent repressive H3K27me3 mark [30] , and the chromatin active H3K4me3 mark were also analysed [3] ( Fig. 5b ). Absence of Bmi1 led to an important increase in H3K27me3 mark bound and significantly enriched for the H2AK119ub signal in the promoter regions of the downregulated CyclinA2, Gbe1 and Gmnn genes, but not in the promoters of upregulated p16 INK4a , Il1 and Tgfβ3 genes in Bmi1 f/f ;αMHC-Cre tg/+ hearts ( Fig. 5b ). However, Bmi1 binding was located at the promoters of downregulated genes in the Bmi1 f/f ;αMHC-Cre +/+ control hearts. Interestingly, mDCM heart cells showed a stronger association with H3K4me3 at the RD domain in the p16 INK4a /ARF locus, which has been demonstrated to be the main Bmi1-binding site in this locus [33] , [34] . In contrast, specific binding of H3K4me3 to the promoter regions of CyclinA2, Gbe1 and Gmnn was lower in the absence of Bmi1 ( Fig. 5b ). These gene expression data strongly correlate with the cardiac phenotype of Bmi1-null mice and suggest the implication of the senescence response in the progression of DCM. CM senescence is increased in a Bmi1-specific manner Sections from 12-week-old Bmi1 f/f ;αMHC-Cre tg/+ hearts, but not controls, stained positive for senescence-associated β-galactosidase (SA-β-gal) marker ( Fig. 6a ). In contrast, apoptotic-mediated caspase 3 expression was not detected in Bmi1 f/f ;αMHC-Cre tg/+ or control hearts ( Fig. 6a ). We next assessed proliferation rate and cardiac SA-β-gal activity [35] in CMs isolated by the Langendorff perfusion method [36] and nonmyocyte subpopulations of FBs (CD3 − /CD31 − /Thy1 + ) and endothelial cells (ECs; CD3 − /CD31 + /Thy1 − ) [37] . Bmi1 expression in Bmi1 f/f ;αMHC-Cre tg/+ CMs was ~10% of the level detected in control CMs, whereas FBs and ECs showed no significant differences between the two genotypes ( Fig. 6b ), as expected [26] . Analysis of the cell-cycle status by 5-bromodeoxyuridine (BrdU) incorporation indicated that total cardiac cells and the FB and EC subpopulations cycled similarly in mutant mice and control littermates ( Fig. 6c ). In Bmi1 fl ;αMHCCre hearts, ~31% of CMs were positive for SA-β-gal activity, compared with 18.4% in control hearts ( Fig. 6d,e ). Surprisingly, ~21% of FBs in Bmi1 -null hearts were also positive, compared with 13% in control hearts ( Fig. 6d,e ), suggesting that CM-expressed Bmi1 might directly control the expression of paracrine factors that spread the senescence response to surrounding populations. To test this, we assessed the contribution of Tgfβ family ligands [17] to DCM in Bmi1 -null mice. Injection of Tgfβ-neutralizing antibodies into Bmi1 f/f ;αMHC-Cre tg/+ mice significantly reduced maximum left ventricular wall thickness and reversed the fractional shortening ( Supplementary Fig. 3c,d ). Moreover, Tgfβ blockade significantly reduced CM cross-sectional area ( Supplementary Fig. 3e ). Together, these results indicate that senescence originating in CMs plays an important role in the development of DCM in Bmi1 -null hearts. 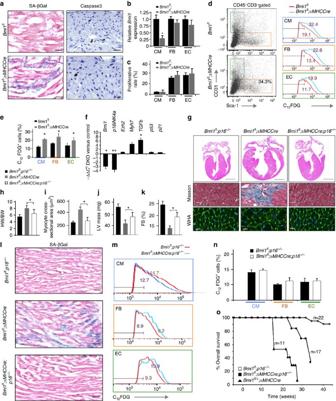Figure 6: Bmi1-mediated cardiomyocyte senescence. (a) Cytochemical staining of SA-β-gal activity and immunostaining of Caspase 3 in paraffin sections of hearts from 15-week-oldBmi1f/f;αMHC-Cretg/+mice andBmi1f/controls. Bars, 50 μm. (b) qRT–PCR analysis ofBmi1mRNA expression in sorted populations of CMs, endothelial cells (ECs) and FBs fromBmi1f/f;αMHC-Cretg/+andBmi1f/mice. Expression is standardized to β-actin and is expressed relative to the level inBmi1f/mice (means±s.d.;n=12, *P<0.05; Student’st-test). (c) Proliferation rate of CM, EC and FB subpopulations measured byin vivoBrdU incorporation over 1 week. Values are means±s.d. (n=5). (d,e) Representative histograms for C12-fluorescein show the relative levels of SA-β-gal in CM, EC and FB subsets fromBmi1f;αMHCCreand control mice (d); the values above the peaks are the median fluorescence intensities of the respective populations. (e) Percentage of SA-β-gal-positive cells in CM, EC and FB subpopulations. Values are means±s.d. (n=6, *P<0.05; Student’st-test). (f) qRT–PCR analysis of the expression ofBmi1,p16INK4a,Ezh2,Myh7,Tgfβ, p53andp21mRNA in total heart cells fromBmi1fl/fl;αMHC-Cretg/+;p16INK4a−/−mice andBmi1fl/fl;αMHC-Cre+/+;p16INK4a−/−mice. Values are means±s.d.;n=10 (**P<0.001, *P<0.05; Student’st-test). (g) The gross cardiac phenotype of 12-week-oldBmi1fl/fl;αMHC-Cre+/+;p16INK4a−/−(Bmi1fl;p16−/−),Bmi1fl/fl;αMHC-Cretg/+;p16INK4a+/+(Bmi1fl;αMHCCre) andBmi1fl/fl;αMHC-Cretg/+;p16INK4a−/−(Bmi1fl;αMHCCre;p16−/−) mice. Representative views are shown of H&E-stained heart cross-sections at the midventricle (bars, 1 mm), Masson’s trichrome staining of left ventricle to detect fibrosis (bars, 40 μm) and WGA staining to outline cardiomyocytes (bars, 10 μm). (h–k) HW/BW ratios (h), myocyte cross-sectional area (i), left ventricular wall thickness (j) and fractional shortening (k) in 12-week-oldBmi1fl;p16−/−,Bmi1fl;αMHCCreandBmi1fl;αMHCCre;p16−/−mice. Data are means±s.d.n=8 mice per group (*P<0.05; Student’st-test). (l) Cytochemical staining of SA-β-gal activity in paraffin sections of hearts fromBmi1fl;p16−/−),Bmi1fl;αMHCCre) andBmi1fl;αMHCCre;p16−/−mice. Scale bars, 50 μm. (m,n) Representative fluorescence histograms show the relative levels of SA-β-gal in CM, EC and FB subsets fromBmi1fl;p16−/−andBmi1fl;αMHCCre;p16−/−hearts (m); the values above the peaks are the median fluorescence intensities of the respective populations. Percentage of SA-β-gal-positive cells in CM, EC and FB subpopulations (n). Values are means±s.d. (n=6; Student’st-test). (o) Kaplan–Meier survival curves forBmi1fl;p16−/−,Bmi1fl;αMHCCreandBmi1fl;αMHC-Cre;p16−/−littermates (means±s.d., **P<0.001; Student’st-test). Figure 6: Bmi1-mediated cardiomyocyte senescence. ( a ) Cytochemical staining of SA-β-gal activity and immunostaining of Caspase 3 in paraffin sections of hearts from 15-week-old Bmi1 f/f ;αMHC-Cre tg/+ mice and Bmi1 f/ controls. Bars, 50 μm. ( b ) qRT–PCR analysis of Bmi1 mRNA expression in sorted populations of CMs, endothelial cells (ECs) and FBs from Bmi1 f/f ;αMHC-Cre tg/+ and Bmi1 f/ mice. Expression is standardized to β-actin and is expressed relative to the level in Bmi1 f/ mice (means±s.d. ; n =12, * P <0.05; Student’s t -test). ( c ) Proliferation rate of CM, EC and FB subpopulations measured by in vivo BrdU incorporation over 1 week. Values are means±s.d. ( n =5). ( d , e ) Representative histograms for C 12 -fluorescein show the relative levels of SA-β-gal in CM, EC and FB subsets from Bmi1 f ;αMHCCre and control mice ( d ); the values above the peaks are the median fluorescence intensities of the respective populations. ( e ) Percentage of SA-β-gal-positive cells in CM, EC and FB subpopulations. Values are means±s.d. ( n =6, * P <0.05; Student’s t -test). ( f ) qRT–PCR analysis of the expression of Bmi1 , p16 INK4a , Ezh2 , Myh7 , Tgfβ, p53 and p21 mRNA in total heart cells from Bmi1 fl/fl ; αMHC-Cre tg/+ ; p16 INK4a −/− mice and Bmi1 fl/fl ; αMHC-Cre +/+ ; p16 INK4a −/− mice. Values are means±s.d. ; n =10 (** P <0.001, * P <0.05; Student’s t -test). ( g ) The gross cardiac phenotype of 12-week-old Bmi1 fl/fl ; αMHC-Cre +/+ ; p16 INK4a −/− ( Bmi1 fl ; p16 −/− ), Bmi1 fl/fl ; αMHC-Cre tg/+ ; p16 INK4a +/+ ( Bmi1 fl ; αMHCCre ) and Bmi1 fl/fl ; αMHC-Cre tg/+ ; p16 INK4a −/− ( Bmi1 fl ; αMHCCre ; p16 −/− ) mice. Representative views are shown of H&E-stained heart cross-sections at the midventricle (bars, 1 mm), Masson’s trichrome staining of left ventricle to detect fibrosis (bars, 40 μm) and WGA staining to outline cardiomyocytes (bars, 10 μm). ( h – k ) HW/BW ratios ( h ), myocyte cross-sectional area ( i ), left ventricular wall thickness ( j ) and fractional shortening ( k ) in 12-week-old Bmi1 fl ; p16 −/− , Bmi1 fl ; αMHCCre and Bmi1 fl ; αMHCCre ; p16 −/− mice. Data are means±s.d. n =8 mice per group (* P <0.05; Student’s t -test). ( l ) Cytochemical staining of SA-β-gal activity in paraffin sections of hearts from Bmi1 fl ; p16 −/− ), Bmi1 fl ; αMHCCre ) and Bmi1 fl ; αMHCCre ; p16 −/− mice. Scale bars, 50 μm. ( m , n ) Representative fluorescence histograms show the relative levels of SA-β-gal in CM, EC and FB subsets from Bmi1 fl ; p16 −/− and Bmi1 fl ; αMHCCre ; p16 −/− hearts ( m ); the values above the peaks are the median fluorescence intensities of the respective populations. Percentage of SA-β-gal-positive cells in CM, EC and FB subpopulations ( n ). Values are means±s.d. ( n =6; Student’s t -test). ( o ) Kaplan–Meier survival curves for Bmi1 fl ; p16 −/− , Bmi1 fl ; αMHCCre and Bmi1 fl ; αMHC-Cre ; p16 −/− littermates (means±s.d., ** P <0.001; Student’s t -test). Full size image Bmi1 limits the senescence response in the heart by repressing Cdkn2a To further define the involvement of senescence in the DCM of cardiac Bmi1-deficient mice, we eliminated p16 INK4a expression in the αMHCCre -mediated Bmi1 -null background, generating Bmi1 fl/fl ; αMHC-Cre tg/+ ; p16 INK4a −/− mice and Bmi1 fl/fl ; αMHC-Cre +/+ ; p16 INK4a −/− littermates. Deletion of p16 INK4a ( p16 −/− ), with p19ARF expression unaffected [38] , was neither accompanied by compensatory upregulation of other Polycomb members nor by increase in p53 and p21 senescence markers ( Fig. 6f ). Moreover, p16 −/− mice with intact Bmi1 ( Bmi1 fl/fl ;p16 −/− ) showed no noticeable adult cardiac abnormalities over the period of study (40 weeks; Fig. 6g–k ). Bmi1 fl/fl ; αMHC-Cre tg/+ ; p16 −/− mice had normal expression levels of the hypertrophy marker Myh7 and the profibrosis factor Tgfβ ( Fig. 6f ), and their hearts were of near normal size ( Fig. 6g,h ) and contained CMs of normal cross-sectional area, with no gross evidence of fibrosis ( Fig. 6g,i ). Bmi1 fl/fl ; αMHC-Cre tg/+ ; p16 −/− mice also had normal left ventricular wall thickness ( Fig. 6j ) and significantly improved FS capacity ( Fig. 6k ). Notably, the deletion of p16 almost completely averted the senescence effect of cardiac Bmi1 deletion, as shown by the normal proportion of CMs exhibiting SA-β-gal activity (14.4% in Bmi1 fl/fl ; αMHC-Cre tg/+ ; p16 −/− mice and 15.2% in Bmi1 fl/fl p16 −/− controls; Fig. 6l–n ). Moreover, p16 deletion significantly improved survival of mice lacking Bmi1 ( Fig. 6n ), suggesting that p16 INK4a is required for the senescence effect in Bmi1-null hearts. Exposure of an old mouse to the circulation of a young mouse by parabiosis can reverse major effects of age-related cardiac hypertrophy [39] . Moreover, senescent cells can communicate with their environment in a paracrine manner [17] . These observations prompted us to examine the impact of the systemic environment on senescence by surgically conjoining the circulation of Bmi1 f/f ; αMHC-Cre tg/+ and control littermate mice in parabiotic pairs ( Fig. 7a ). Efficiency of parabiosis was evaluated by using congenic markers to distinguish blood cells in parabiotic pairs, in which one partner was CD45.1 + ( Supplementary Fig. 3f ). The effect of a wild-type circulation on DCM hearts (parabiotic no-DCM/DCM pairs) after 1 month was readily apparent on cardiac histologic sections ( Fig. 7b ). Masson’s trichrome staining showed a reduction in interstitial cardiac fibrosis in the DCM heart, accompanied by reduced CM size ( Fig. 7b ). Accordingly, parabiosis reduced the HW/BW ratio and CM cross-sectional area in the DCM heart, whereas isochronic parabiosis (no-DCM/no-DCM or DCM/DCM pairs) had no effect ( Fig. 7c,d ). Parabiotic exposure of DCM mice to the circulation of healthy non-DCM littermates for 4–5 weeks rescued FS from initial values of 16.0±1.1–24.0±2.4% ( Fig. 7e ), indicating that the wild-type circulation restores cardiac function of the DCM partner in no-DCM/DCM pairs. These data indicate that factors in the circulation could modify discrete molecular pathways associated with ventricular remodelling and DCM, allowing reversal of the dilated cardiac function. Remarkably, however, DCM-related paracrine senescence factors were not able to transmit the DCM phenotype to healthy mice. 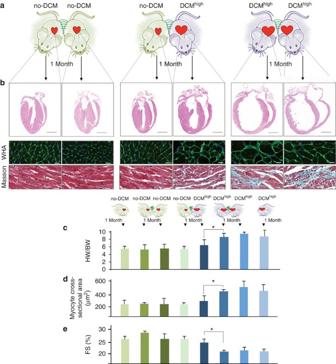Figure 7: Paracrine senescence response of Bmi1-related DCM does not transmit to healthy mice. (a) Parabiotic pairings; no-DCM asBmi1flmice and DCMhighasBmi1fl/fl;αMHC-Cremice. Comparisons were always made with littermate pairs (no-DCM to no-DCM or DCMhighto DCMhigh). (b) The gross cardiac phenotype of 12-week-old mice after 4 weeks of parabiosis as indicated. Representative views are shown of H&E-stained cross-sections at the midventricle (bars, 1 mm), Masson’s trichrome staining of left ventricle to detect fibrosis (bars, 40 μm), and WGA staining to outline cardiomyocites (bars, 10 μm). (c–e) HW/BW ratio (c), myocyte cross-sectional area (d) and fractional shortening (e) after 4 weeks of parabiosis as indicated. Data are means±s.d.;n=8 mice per group (*P<0.05; Student’st-test). Figure 7: Paracrine senescence response of Bmi1-related DCM does not transmit to healthy mice. ( a ) Parabiotic pairings; no-DCM as Bmi1 fl mice and DCM high as Bmi1 fl/fl ; αMHC-Cre mice. Comparisons were always made with littermate pairs (no-DCM to no-DCM or DCM high to DCM high ). ( b ) The gross cardiac phenotype of 12-week-old mice after 4 weeks of parabiosis as indicated. Representative views are shown of H&E-stained cross-sections at the midventricle (bars, 1 mm), Masson’s trichrome staining of left ventricle to detect fibrosis (bars, 40 μm), and WGA staining to outline cardiomyocites (bars, 10 μm). ( c – e ) HW/BW ratio ( c ), myocyte cross-sectional area ( d ) and fractional shortening ( e ) after 4 weeks of parabiosis as indicated. Data are means±s.d. ; n =8 mice per group (* P <0.05; Student’s t -test). Full size image Here we propose a mechanistic model of how Bmi1 protects from DCM by limiting heart senescence. Absence of cardiac Bmi1 profoundly compromises expression of the senescence marker p16 INK4a in CMs, leading to a cardiac-senescent response caused likely by SASP, which mobilizes the systemic and local tissue milieu for tissue repair and aging [12] , [40] . The detection of senescence factors by neighbouring healthy cells might further drive cellular senescence, thus contributing to a spiral of increasing inflammation and dysfunction that increases the original features of the DCM. The increasing burden of senescent cells might contribute to the early aetiology of DCM and accelerate progression of these age-related cardiac diseases ( Fig. 8a ). Remarkably, this paracrine nonproliferative senescence phenotype is not propagated between organisms via parabiosis, whereas a healthy circulation is able to reverse CM hypertrophy in mice with DCM. This effect is gender-independent and the reduction in CM size translates into a reduction in global cardiac mass. Factors present in the circulation of healthy mice are thus to some extent able to reverse critical structural and molecular aspects of cardiac aging. Although the full cast of factors involved in the rejuvenation of DCM are yet to be identified, our data provide proof of principle that signals from the systemic environment can override age-related, intrinsic changes in DCM, suggesting that these changes are predominantly epigenetic. In fact, in recent years, emerging evidence indicates that there are factors within the blood of young animals that have the ability to restore youthful characteristics to a number of organ systems in older animals [39] , [41] . These studies offer compelling evidence that effects of aged-associated disease can be reversed. 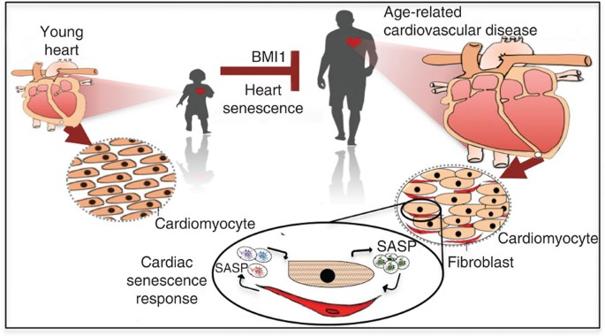Figure 8: A model for the impact of cardiac-specific Bmi1 action. (a) As aging poses the largest risk for cardiovascular disease, the cardiac Bmi1 action could be determinant to limit the heart senescence response. Our data establish the idea that the nonproliferative cardiomyocyte-related senescence phenotype can be locally propagated through the SASP. Figure 8: A model for the impact of cardiac-specific Bmi1 action. ( a ) As aging poses the largest risk for cardiovascular disease, the cardiac Bmi1 action could be determinant to limit the heart senescence response. Our data establish the idea that the nonproliferative cardiomyocyte-related senescence phenotype can be locally propagated through the SASP. Full size image Risk assessment in DCM patients is currently limited to echocardiography studies, measurement of haemodynamic parameters and cardiopulmonary exercise performance. Understanding the role of epigenetic regulators in adult cardiac senescence provides a possible route towards more accurate profiling of cardiac dysfunction in dilated cardiomyopathies. Modulation of cardiac senescence response may further provide a novel strategy for treating heart failure, with Bmi1 serving as an attractive target. Mice ckoBmi1 fl/+ mice [24] were backcrossed to the C57BL/6 background. Mice used in this study included αMHC-Cre tg/+ (ref. 26 ), αMHC TM -Cre tg/+ (ref. 27 ), Nkx2.5-Cre tg/+ (ref. 25 ), MLC2-rRTA tg/+ (ref. 28 ) and p16 INK4a −/− (ref. 38 ). The αMHC-Cre tg/+ and αMHC TM -Cre tg/+ lines were kindly provided by Dr Redondo, Nkx2.5-Cre tg/+ by Dr de la Pompa, MLC2-rRTA tg/+ by Dr Lara-Pezzi and p16 INK4a −/− by Dr Berns. For the generation of tetO-Bmi1 tg/+ mice, Bmi1 cDNA was cloned into the pBS31 vector that included the minimal tetracycline-independent promoter. This Bmi1 vector was coelectroporated together with the vector harbouring FLPe recombinase under the control of the CAGGS promoter into KH2 ES cells (Open Biosystems). All genotyping primers are listed in Supplementary Table 1 . All strains were on the C57BL/6J background; male and female mice aged 5–12 weeks were used, in the cases of not indicated. For iBmi1 tg/tg ;MLC2 tg/+ and control mice, doxycycline (2 mg ml −1 , supplemented with sucrose at 5 mg ml −1 ) was administrated to mice in drinking water for 2 weeks). The αMHC TM -Cre line and their control littermates were injected with 1 mg TM (Sigma) in corn coil on five consecutive days. All mice were bred in-house in a pathogen-free environment and were provided with standard care and nutrition according to the EU guidelines. All animal study proposals were approved by the Centro Nacional de Investigaciones Cardiovasculares (CNIC). For cardiogenesis studies, hearts at various embryonic stages or post-natal (P) days were collected for RNA/protein analysis or for histology. Echocardiography and MRI Echocardiograms were performed on mice anaesthetized with 2.0% isoflurane, using a Vevo 770 High-Resolution In Vivo Micro-Imaging System and RMV 707B Scanhead (VisualSonics Inc). Scans were conducted by two experienced researchers blinded to the mouse genotype. Measurements of left parasternal long and short axes and M-mode (left parasternal short axis) images were obtained at a heart rate of 500–550 bpm. LV end-diastolic diameter (LVEDD), LV end-systolic diameter (LVESD) and wall thickness were measured from M-mode tracings, and the average of three consecutive cardiac cycles is reported. The LV fractional shortening percentage was calculated as ([LVEDD−LVESD]/LVEDD) × 100 MRI of lung was performed with a 7-T Agilent scanner (Agilent, Santa Clara, USA) equipped with a DD2 console and an actively shielded gradient set (205/120 insert of maximum 130 mT m −1 gradient strength). For image acquisition, we employed a combination of volume coil/surface coil coil to enhance signal-to-noise ratio formed by a 72-mm inner diameter quadrature birdcage TX coil (Rapid Biomedical GmBH, Germany) and an actively detuning 30-mm flexible customized surface RX coil (Neos Biotec, Pamplona, Spain). Following a tripilot gradient-echo image, a gradient-echo sequence without gating was used to acquire oblique coronal slices (one to two slices) and axial slices (7–10 slices covering the entire lung, 72-s acquisition time per slice) using the following parameters: TR/TE=6.7/2.2 ms, flip angle=10 degree, bandwidth=100 kHz, field of view=3 × 3 cm, matrix=256 × 128, slice thickness=1 mm and number average experiment (Number average EXperiments=60). Mice were anaesthetized with 2% isoflurane and oxygen and positioned on a thermoregulated (38.7 °C) mouse bed. Ophthalmic gel was placed in their eyes to prevent retinal drying. Human DCM samples The study population comprised six patients with medically refractory DCM, excluding specifically those patients with the evidence of ischaemic cardiomyopathy or myocarditis. Before cardiac transplantation, patients received a two-stage drug regime designed to avoid deterioration (β1/β2-blocker (carvedilol), angiotensin-converting enzyme inhibitor (lisinopril), angiotensin receptor I antagonist (losartan) and aldosterone antagonist (spironolactone)). Patients were subsequently switched to a selective β1 blocker (bisoprolol) and given the β2-agonist, clenbuterol, with a view to stimulate hypertrophy and improve cardiac function. Echocardiography and exercise testing were performed regularly during treatment before transplantation to monitor the recovery process. In addition, four ventricular samples were available for mRNA analysis from donor organs used for transplantation ( n =2), and donor organs unsuitable for transplantation ( n =2). Data collected from these RNA samples were used in gene expression analyses. Histology and immunohistochemical analyses For histological analysis, embryos or heart tissues were fixed in 10% paraformaldehyde (PFA) at the stages indicated in each figure legend, dehydrated and embedded in paraffin for preparation of 5- or 10-μm histological sections. Rehydrated slides were stained with haematoxylin and eosin and Masson’s trichrome. For determination of CM cross-sectional area, deparaffinized and rehydrated heart sections were incubated for 1 h at room temperature with fluorescein isothiocyanate (FITC)-labelled wheatgerm agglutinin (Sigma-Aldrich) to visualize myocyte membranes. Regions that included the circular shapes of capillaries were selected from the epicardial side of the LV-free walls. The mean cross-sectional area of CMs was determined from 60 to 80 cells. For fluorescence detection of SA-β-gal activity, cells (10 7 cell ml −1 ) were incubated with C 12 FDG (fluorescein di-β- D -galactopyranoside; 33 μM; Sigma), a β-galactosidase substrate that generates a fluorescent product upon cleavage, for 60 min at 37 °C (ref. 35 ). Cytochemical detection of senescent cells in vitro was determined in cells and fixed tissues with the Senescence β-Galactosidase Staining Kit (Cell Signaling). Chromatin immunoprecipitation (ChIP) assays For ChIP analysis, we used sorted 10 6 cells per condition and added formaldehyde directly to the tissue culture medium to a final concentration of 1% and incubated cultures for 10 min at room temperature on a shaking platform. We stopped the crosslinking by adding glycine to a final concentration of 0.125 M. We washed crosslinked cells twice with cold phosphate-buffered saline and lysed them at a density of 5 × 10 6 cells ml −1 for 10 min at 4 °C in 1% SDS, 50 mM Tris-HCl (pH 8.0) and 10 mM EDTA-containing protease inhibitors. We sonicated lysates to obtain chromatin fragments <1 kb and centrifuged them for 15 min in a microfuge at room temperature. We diluted 400 μl of lysate 1:10 with 1.1% Triton-X100, 2 mM EDTA, 150 mM NaCl and 20 mM Tris-HCl (pH 8.0) containing protease inhibitors, precleared with 50% salmon sperm DNA and protein A agarose slurry (Upstate). Antibodies used for ChIP assays [42] were rabbit polyclonal anti-Bmi1, H3K27me3, H2AK119 and H3K4me3 (all from Upstate; 1:2,500). We then added salmon sperm DNA and protein A agarose beads (60 μl) and incubated for 1 h. We washed the immunoprecipitated pellets with 0.1% SDS, 1% Triton-X100, 2 mM EDTA, 20 mM Tris-HCl (pH 8.0) and 150 mM NaCl (one wash); 0.1% SDS, 1% Triton-X100, 2 mM EDTA, 20 mM Tris-HCl (pH 8.0) and 500 mM NaCl (one wash); 0.25 M LiCl, 1% Nonidet P-40, 1% sodium deoxycholate, 1 mM EDTA and 10 mM Tris-HCl, pH 8.0 (one wash); and 10 mM Tris-HCl (pH 8.0) and 1 mM EDTA (two washes). We then eluted the chromatin from the beads twice by incubation with 250 μl 1% SDS and 0.1 M NaHCO 3 during 15 min at room temperature with rotation. After adding 20 μl of 5 M NaCl, we reversed the crosslinks for 4 h at 65 °C. Samples were supplemented with 20 μl of 1 M Tris-HCl (pH 6.5), 10 μl of 0.5 M EDTA, 20 μg of RNase A and 40 μg of proteinase K and incubated for 1 h at 45 °C. DNA from precipitated complexes was amplified using reverse transcription–polymerase chain reaction (RT–PCR). RT–PCR amplifications were performed in triplicate with multiple dilutions, and primer sequences are included in the Supplementary Table 1 . RNA extraction and real-time PCR Heart tissue samples were stored in RNAlater RNA stabilization reagent (QIAGEN) at 4 °C. Total RNA was extracted using the RNeasy Fibrous Tissue Mini Kit (QIAGEN). First-strand cDNA synthesis was performed with 1 μg of total RNA, random hexamers and SuperScript III Reverse Transcriptase (Invitrogen). Real-time PCR was performed using a QuantiTect SYBR Green PCR kit (QIAGEN) in a Light-Cycler (Roche). The expression level of each gene was normalized to that of 18S rRNA, which served as an endogenous internal control. The primer sequences are available at the Supplementary Table 1 . Cardiac hypertrophy induction Isoproterenol (60 mg per kg body weight) was administered to 9-week-old mice for 14 days using subdermally implanted ALZET osmotic minipumps. PBS-filled minipumps were used as a control. For TAC surgery, mice (8–10 weeks old, 21–24 g body weight) were anaesthetized by intraperitoneal injection of a mixture of xylazine (5 mg kg −1 ) and ketamine (100 mg kg −1 ). The animals were then placed in a supine position, an endotracheal tube was inserted and the animals were ventilated using a volume-cycled rodent ventilator with a tidal volume of 0.4 ml room air and a respiratory rate of 110 breaths per minute. The chest cavity was exposed by cutting open the proximal portion of the sternum. The aortic arch between the innominate and left common carotid arteries was isolated and was constricted with a 7–0 nylon suture tied firmly three times against a 25-gauge blunted needle for LI-TAC or a 27-gauge needle for HI-TAC. Sham-operated mice underwent the same surgical procedure, including isolation of the aorta, but without placement of the suture. Tgf-β blocking activity assay DCM mice ( Bmi1 fl α MHC-Cre tg/+ ) received intraperitoneal injections of Tgf-β antibody (10 mg per kg body weight in PBS; AB-100-NA; R&D Systems) every 3 days for 2 weeks before being killed. Control mice were treated with identical doses of rabbit IgG (R&D Systems). Protein analysis Antibodies used for western blots were as follows: anti-Bmi1 (Millipore), anti-Ezh2 (Active Motif), anti-aMHC (Millipore), anti-H3K9me3 (Upstate), anti-murine p16 (Santa Cruz Biotechnology), anti-human p16 (Cell Signaling) and anti-β-actin (Sigma; these antibodies were used at 1:500). Secondary antibody was the horseradish peroxidase-linked anti-mouse IgG (Dako; 1:2,500). Isolation of CMs and cardiac FBs Cells were isolated from Langendorff heart preparations followed by enzymatic digestion [43] . For isolation of nonmyocyte-enriched cells, hearts were dissected free of vessels and atria, washed in ice-cold modified Krebs–Henseleit bicarbonate buffer (pH 7.2; Sigma-Aldrich) and rapidly cut into pieces. The heart pieces were incubated in 5 ml of digesting solution (0.25 mg ml −1 Liberase TH (Roche) and 10 mM HEPES in balanced salt solution-containing calcium and magnesium) for 8 min at 37 °C with vigorous stirring. The supernatant was then added to 10 ml of ice-cold Krebs–Henseleit bicarbonate. Five millilitres of fresh digesting solution were added to the remaining tissue fragments, and the digestion and sampling steps were repeated until all the tissues were dissolved. The collected cells were filtered through a 35-μm nylon mesh (BD Falcon) and then used for flow cytometry. Different cellular subsets were incubated with phycoerythrin-conjugated anti-Thy1 antibody (eBioscience), FITC-conjugated anti-CD31 antibody (BD Biosciences) and allophycocyanin-conjugated CD3 antibody (eBioscience), after which they were analysed and sorted on a FACSAria II flow cytometer (BD Biosciences) using the FlowJo softwarem (these antibodies were used at 1:100). For analysis of SA-β-gal expression, cells were stained with the fluorogenic β-galactosidase substrate fluorescein di-β- D -galactopyranoside (1:250). Cell proliferation BrdU (Sigma-Aldrich) was injected daily into the peritoneum (100 mg per kg body weight in PBS) for 3 days, with the last injection 2 h before harvesting the hearts. The hearts were fixed in 4% PFA, paraffin-embedded and sectioned. BrdU-positive nuclei were detected with mouse monoclonal anti-BrdU primary antibody (Dako; 1:250) and immunofluorescent staining as described above. BrdU- or Ki67-labelled cells and 4',6-diamidino-2-phenylindole (DAPI)-stained nuclei were counted in nonmyocyte cells from 5 to 10 fields ( × 400 magnification) with focal fibrosis and/or expanded interstitium (identified with wheatgerm agglutinin staining) and in areas with preserved myocardial architecture (for example, absence of both focal fibrosis and expanded interstitium) in 9–15 sections per heart. Myocytes were identified with fluorescent microscopy visualization of sarcomeres. Nuclei of sarcomere-negative cells within interstitial regions were designated as nonmyocyte nuclei. Nuclei were quantified using the ImageJ nucleus counter software. The percentage of proliferating cells was calculated as the number of positive BrdU- or Ki67-labelled nuclei divided by the number of DAPI-stained nuclei. Parabiosis Anaesthetized mice were shaved at the corresponding lateral aspects and matching skin incisions were made from the olecranon to the knee joint of each mouse, and the subcutaneous fascia was bluntly dissected to create ~0.5 cm of free skin. The olecranon and knee joints were attached by a single 5–0 polypropylene suture and tie, and the dorsal and ventral skins were approximated by continuous suture. A single dose of flunixin meglumine (Schering-Plough, 1 mg kg −1 ) was injected subcutaneously into each partner at the end of the surgical procedure. One month after surgery, blood samples were obtained from each of the partners for analysis of haematopoietic progenitors. Statistical analysis All data are expressed as the mean±s.d. Paired data were evaluated using Student’s t -test. Survival rates among mice were analysed using the long-rank test. Differences were considered statistically significant at P <0.05. Accession codes : The RNAseq data from mDCM and hDCM samples have been deposited in the Gene Expression Omnibus under accession code GSE64391 and GSE65447, respectively How to cite this article: Gonzalez-Valdes, I. et al. Bmi1 limits dilated cardiomyopathy and heart failure by inhibiting cardiac senescence. Nat. Commun. 6:6473 doi: 10.1038/ncomms7473 (2015).